LSD1 promotes oxidative metabolism of white adipose tissue Exposure to environmental cues such as cold or nutritional imbalance requires white adipose tissue (WAT) to adapt its metabolism to ensure survival. Metabolic plasticity is prominently exemplified by the enhancement of mitochondrial biogenesis in WAT in response to cold exposure or β3-adrenergic stimulation. Here we show that these stimuli increase the levels of lysine-specific demethylase 1 (LSD1) in WAT of mice and that elevated LSD1 levels induce mitochondrial activity. Genome-wide binding and transcriptome analyses demonstrate that LSD1 directly stimulates the expression of genes involved in oxidative phosphorylation (OXPHOS) in cooperation with nuclear respiratory factor 1 (Nrf1). In transgenic (Tg) mice, increased levels of LSD1 promote in a cell-autonomous manner the formation of islets of metabolically active brown-like adipocytes in WAT. Notably, Tg mice show limited weight gain when fed a high-fat diet. Taken together, our data establish LSD1 as a key regulator of OXPHOS and metabolic adaptation in WAT. Lysine-specific demethylase 1 (LSD1) selectively removes mono- and dimethyl groups from lysine 4 or lysine 9 of histone H3, thereby causing either repression or activation of gene transcription [1] , [2] . LSD1 is ubiquitously expressed and essential for early embryonic development, as knockout mice die before day E7.5 (refs 3 , 4 , 5 , 6 ). In various types of cancer, LSD1 expression is increased compared with normal tissue and has been correlated with malignancy or metastatic potential of tumours [1] , [7] , [8] . Although these observations indicate the necessity to control LSD1 expression, physiological effects of altered LSD1 levels have not been investigated in vivo . Knockdown of LSD1 in 3T3-L1 cells has recently been reported to result in impaired differentiation [9] or altered oxidative capacities [10] , hinting at potential physiological roles of LSD1 in the control of adipogenesis and metabolic processes in organs such as adipose tissue. Adipose tissue is an important metabolic regulator of energy balance [11] . The major types of adipose tissue in mammals are white adipose tissue (WAT) and brown adipose tissue (BAT). Unilocular WAT is mainly located in the abdominal and subcutaneous areas and is highly adapted to store excess energy in the form of triglycerides. Conversely, multilocular BAT is predominantly located in the interscapular area and characterized by a high content of mitochondria and the expression of uncoupling protein 1 (Ucp1) [12] , [13] . Ucp1 expression results in the production of heat in a process called non-shivering or adaptive thermogenesis [11] , [14] . Appearance of a third type of fat cells, termed brown-like or beige adipocytes, has been observed in white fat depots in response to cold exposure or β3-adrenergic stimulation [15] , [16] , [17] . This cell type shares common characteristics with brown adipocytes, including increased mitochondria number and activity [18] . Oxidative phosphorylation (OXPHOS) and mitochondrial biogenesis have been shown to be regulated by nuclear respiratory factor 1 (Nrf1) and transcription factor A, mitochondrial (Tfam) [19] , [20] , [21] , [22] . Here we show that cold exposure or β3-adrenergic stimulation of mice increases LSD1 levels in WAT. Mechanistic studies unravel that elevated LSD1 levels are sufficient to promote OXPHOS in adipocytes. Furthermore, we demonstrate that LSD1 cooperates with Nrf1 to promote expression of genes involved in mitochondrial biogenesis and cellular oxidative function. In mice, transgenic expression of LSD1 promotes the formation of islets of functional brown-like adipocytes in WAT, which limits weight gain and type-2 diabetes in response to a high-fat diet. Taken together, our data establish LSD1 as a regulator of OXPHOS and metabolic adaptation of WAT. Cold and β3-adrenergic signalling increase LSD1 levels Cold exposure of mice has been shown to enhance thermogenic and oxidative capacities of WAT via β3-adrenergic signalling [17] , [18] , [23] . When analysing previously deposited gene expression data [18] of C57/Bl6 mice treated with the β3-adrenergic agonist CL316,243, we noticed that LSD1 mRNA levels were upregulated in epididymal (ep) WAT ( Supplementary Fig. 1a ). To investigate a potential function of LSD1 in thermogenic or oxidative adaptation of WAT, we exposed C57/Bl6 mice to cold or treated them with CL316,243. LSD1 protein was significantly increased in inguinal (ing) WAT and epWAT of cold-exposed mice ( Fig. 1a and Supplementary Fig. 1b ). Similarly, we observed elevated LSD1 protein levels in ingWAT of mice treated with CL316,243 ( Fig. 1b ). In quantitative reverse-transcription PCR (qRT–PCR) analyses, we found upregulation of transcript levels of LSD1 and thermogenic markers (Prdm16, Pgc-1α and Ucp1) on CL316,243 treatment ( Supplementary Fig. 1c ). 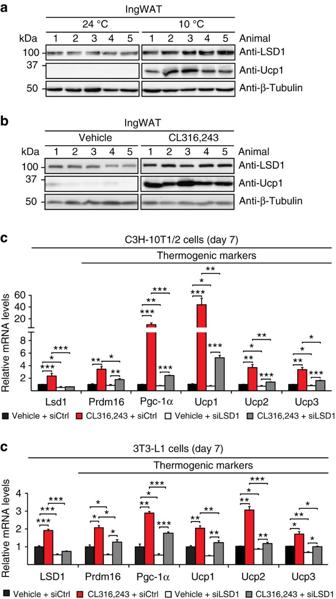Figure 1: LSD1 expression is induced in white fat pads after cold exposure or β3-adrenergic treatment of mice. Western blot analysis of LSD1 and Ucp1 in inguinal (ing) WAT of mice (a) maintained at either 24 or 10 °C, or (b) treated with vehicle or the β3-adrenergic agonist CL316,243. β-Tubulin was used as a loading control. Relative transcript levels of the indicated markers in differentiated (day 7) (c) C3H-10T1/2 or (d) 3T3-L1 cells treated with vehicle or CL316,243 and transfected with unrelated control siRNA (siCtrl) or siRNA directed againstLSD1(siLSD1).a,b:n=10;c,d:n=9; s.d. represents+s.e.m. Experiments (c,d) were independently repeated at least three times in triplicate. Statistical analysis was performed using two-tailed Student’st-test. *P<0.05, **P<0.01 and ***P<0.001. Figure 1: LSD1 expression is induced in white fat pads after cold exposure or β3-adrenergic treatment of mice. Western blot analysis of LSD1 and Ucp1 in inguinal (ing) WAT of mice ( a ) maintained at either 24 or 10 °C, or ( b ) treated with vehicle or the β3-adrenergic agonist CL316,243. β-Tubulin was used as a loading control. Relative transcript levels of the indicated markers in differentiated (day 7) ( c ) C3H-10T1/2 or ( d ) 3T3-L1 cells treated with vehicle or CL316,243 and transfected with unrelated control siRNA (siCtrl) or siRNA directed against LSD1 (siLSD1). a , b : n =10; c , d : n =9; s.d. represents+s.e.m. Experiments ( c , d ) were independently repeated at least three times in triplicate. Statistical analysis was performed using two-tailed Student’s t -test. * P <0.05, ** P <0.01 and *** P <0.001. Full size image To determine whether upregulation of LSD1 in response to physiological stimuli results in altered properties of white adipocytes, we analysed C3H-10T1/2 multipotent mesenchymal cells and 3T3-L1 preadipocytes, which both can be differentiated into mature adipocytes by exposure to differentiation medium for 7 days. In accordance with our observations in mice, LSD1 transcript and protein levels were increased in differentiated C3H-10T1/2 and 3T3-L1 adipocytes (day 7) treated with CL316,243 compared with vehicle-treated cells ( Fig. 1c,d and Supplementary Fig. 1d,e ). Thus, LSD1 protein is induced in C3H-10T1/2 and 3T3-L1 adipocytes, and in WAT of mice on cold exposure or by β3-adrenergic signalling. Notably, induction of thermogenic markers [17] , [24] was impaired on short interfering RNA (siRNA)-mediated LSD1 knockdown ( Fig 1c,d and Supplementary Fig. 1d,e ), suggesting that LSD1 mediates β3-adrenergic-induced thermogenesis. LSD1 enhances oxidative capacities of mature adipocytes To determine the genome-wide binding pattern of LSD1, we transduced 3T3-L1 and C3H-10T1/2 preadipocytes with control virus (Ctrl) or lentivirus driving expression of Flag-tagged LSD1 ( Supplementary Fig. 2a,b ). Cells were then subjected to chromatin immunoprecipitation (ChIP) followed by massive parallel sequencing (ChIP-seq). The ChIP-seq analysis of 3T3-L1(Ctrl) and C3H-10T1/2(Ctrl) cells differentiated for 7 days into mature adipocytes revealed 8,303 and 11,659 LSD1 peaks, of which the majority was located at the promoter of 6,904 and 7,048 genes, respectively ( Fig. 2a,b and Supplementary Fig. 2c ). Only 38 and 405 genes, respectively, with LSD1 peaks at promoter were observed in 3T3-L1 and C3H-10T1/2 cells treated with siRNA to induce LSD1 knockdown, thus confirming specificity of the LSD1 antibody ( Supplementary Fig. 2d,e ). In LSD1-overexpressing 3T3-L1(LSD1) and C3H-10T1/2(LSD1) cells, the number of peaks reached 27,221 and 43,903, with 43% and 27% located at the promoter of 9,840 and 8,960 genes, respectively ( Fig. 2a,b and Supplementary Fig. 2c ). We found that the majority of genes targeted by LSD1 in 3T3-L1(Ctrl) cells were also occupied by LSD1 in C3H-10T1/2(Ctrl) cells (70%, Supplementary Fig. 2f ). A comparable overlap was observed for 3T3-L1(LSD1) and C3H-10T1/2(LSD1) cells (85%, Supplementary Fig. 2g ), showing that LSD1 is recruited to similar promoters in both cell lines. Pathway analysis of genes occupied by LSD1 in Ctrl and LSD1-overexpressing cells unravelled ‘adipogenesis’, ‘electron transport chain’, ‘tricarboxylic acid cycle’ and ‘OXPHOS’ ( Fig. 2a–d ). Similarly, for genes only occupied in 3T3-L1(LSD1) or in C3H-10T1/2(LSD1) cells, ‘electron transport chain’ was also identified as significantly enriched pathway ( Fig. 2e,f ). These data demonstrate that LSD1 targets similar sets of genes in 3T3-L1 and C3H-10T1/2 cells. 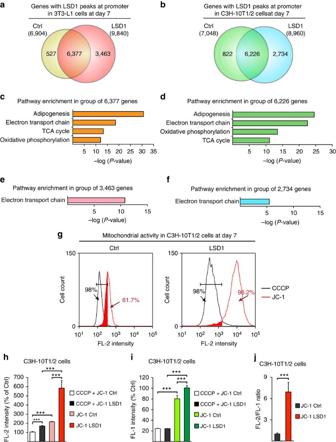Figure 2: LSD1 positively regulates OXPHOS in mature adipocytes. Venn diagram showing the number of genes with LSD1 peaks at promoter in differentiated (day 7) (a) 3T3-L1(Ctrl) and 3T3-L1(LSD1) or (b) C3H-10T1/2(Ctrl) and C3H-10T1/2(LSD1) cells. (c–f) Enriched pathways obtained from GO term analyses for the indicated sets of genes. (g) Mitochondrial activity in differentiated C3H-10T1/2(Ctrl) and C3H-10T1/2(LSD1) cells reflected by red fluorescent JC-1 aggregates (FL-2). Black curves represent the background staining obtained after treatment of samples with the mitochondrial membrane potential disrupter CCCP. Numbers in red show the percentage of cells with increased mitochondrial activity. (h) Relative mitochondrial activity determined by red fluorescence intensity of JC-1 aggregates (FL-2) and (i) relative mitochondrial mass determined by green fluorescence intensity of JC-1 aggregates (FL-1) in C3H-10T1/2(Ctrl) and C3H-10T1/2(LSD1) cells at day 7 of differentiation. Samples treated with CCCP represent background staining. (j) Ratio of mitochondrial activity (FL-2) relative to mitochondrial mass (FL-1) in C3H-10T1/2(Ctrl) and C3H-10T1/2(LSD1) cells at day 7 of differentiation. (g–i):n=6; s.d. represents+s.e.m. Experiments (g–i) were independently repeated at least three times in triplicate. Statistical analysis was performed using (c–f) HOMER analysis or (h–j) two-tailed Student’st-test. ***P<0.001. Figure 2: LSD1 positively regulates OXPHOS in mature adipocytes. Venn diagram showing the number of genes with LSD1 peaks at promoter in differentiated (day 7) ( a ) 3T3-L1(Ctrl) and 3T3-L1(LSD1) or ( b ) C3H-10T1/2(Ctrl) and C3H-10T1/2(LSD1) cells. ( c – f ) Enriched pathways obtained from GO term analyses for the indicated sets of genes. ( g ) Mitochondrial activity in differentiated C3H-10T1/2(Ctrl) and C3H-10T1/2(LSD1) cells reflected by red fluorescent JC-1 aggregates (FL-2). Black curves represent the background staining obtained after treatment of samples with the mitochondrial membrane potential disrupter CCCP. Numbers in red show the percentage of cells with increased mitochondrial activity. ( h ) Relative mitochondrial activity determined by red fluorescence intensity of JC-1 aggregates (FL-2) and ( i ) relative mitochondrial mass determined by green fluorescence intensity of JC-1 aggregates (FL-1) in C3H-10T1/2(Ctrl) and C3H-10T1/2(LSD1) cells at day 7 of differentiation. Samples treated with CCCP represent background staining. ( j ) Ratio of mitochondrial activity (FL-2) relative to mitochondrial mass (FL-1) in C3H-10T1/2(Ctrl) and C3H-10T1/2(LSD1) cells at day 7 of differentiation. ( g – i ): n =6; s.d. represents+s.e.m. Experiments ( g – i ) were independently repeated at least three times in triplicate. Statistical analysis was performed using ( c – f ) HOMER analysis or ( h – j ) two-tailed Student’s t -test. *** P <0.001. Full size image Next, 3T3-L1(Ctrl) and 3T3-L1(LSD1) cells were subjected to global transcriptome analysis (RNA-seq). RNA-seq analysis identified 5,765 genes differentially expressed between 3T3-L1(LSD1) and 3T3-L1(Ctrl) cells at day 7 ( Supplementary Fig. 2h ). Out of these genes, 2,719 were occupied by LSD1 in both, 3T3-L1(LSD1) and 3T3-L1(Ctrl) cells (group 1, Supplementary Fig. 2h ), whereas 1,372 were only occupied in 3T3-L1(LSD1) cells (group 2, Supplementary Fig. 2h ). Pathway analysis for group 1 unravelled ‘adipogenesis’, ‘electron transport chain’, ‘tricarboxylic acid cycle’ and ‘OXPHOS’ ( Supplementary Fig. 2i ). In group 2, ‘electron transport chain’ and ‘OXPHOS’ were also identified as significantly enriched pathways ( Supplementary Fig. 2j ). These observations suggest that in control cells, LSD1 targets genes essential for adipocyte metabolism, and that on increased expression, LSD1 targets additional OXPHOS genes. Notably, in 3T3-L1(LSD1) adipocytes, LSD1 occupies the promoter of and positively regulates almost all (90%) genes of the mitochondrial electron transport chain ( Supplementary Data 1 and Supplementary Fig. 3a,b ). Upregulation of representative OXPHOS genes was confirmed by qRT–PCR analysis in 3T3-L1(LSD1) and C3H-10T1/2(LSD1) cells ( Supplementary Fig. 3c,d ). In addition, LSD1 also targets and increases the transcript levels of the key transcription factor that controls mitochondrial DNA transcription and replication Tfam, and of the main inducers of thermogenesis and oxidative metabolism, including Pgc-1α, Pgc-1β and uncoupling proteins ( Supplementary Fig. 4 ). Together, these data demonstrate that elevated LSD1 levels are sufficient to promote expression of genes involved in OXPHOS and thermogenesis in differentiated adipocytes. Comparison of LSD1 promoter occupancy in 3T3L1(Ctrl) cells at days 0 and 7 of differentiation revealed that 4,671 out of 6,904 genes (68%) only become LSD1 targets in differentiated adipocytes ( Supplementary Fig. 5a ). Interestingly, most of the genes occupied in 3T3-L1(Ctrl) cells at day 7 are already associated with LSD1 in 3T3-L1(LSD1) cells at day 0 (5,689 out of 6,904 genes (82%); Supplementary Fig. 5a ). Thus, LSD1 promoter occupancy in undifferentiated 3T3-L1(LSD1) cells at day 0 resembles that in differentiated 3T3-L1(Ctrl) cells at day 7. Importantly, a large number of these genes (2,406 out of 5,689, group 3) is differentially expressed between 3T3-L1(LSD1) and 3T3-L1(Ctrl) adipocytes at day 7 of differentiation ( Supplementary Fig. 5b ), suggesting that elevated LSD1 levels result in premature occupancy and increased expression of metabolic genes on adipogenic medium ( Supplementary Fig. 5c,d ). Next, we compared the oxidative capacities of differentiated adipocytes by JC-1 assay for mitochondrial content and activity. Elevated LSD1 levels in C3H-10T1/2 and 3T3-L1 cells significantly increased respiratory activity indicated by FL-2 intensity ( Fig. 2g,h and Supplementary Fig. 5e,f ). Higher FL-1 intensity revealed an augmentation in mitochondrial mass ( Fig. 2i and Supplementary Fig. 5g ). The increased ratio between FL-2 and FL-1 for differentiated C3H-10T1/2(LSD1) and 3T3-L1(LSD1) adipocytes demonstrated enhanced mitochondrial activity ( Fig. 2j and Supplementary Fig. 5h ). Thus, in accordance with our RNA-seq data, JC-1 assays show that increased LSD1 expression suffices to induce mitochondrial activity in differentiated adipocytes. LSD1 regulates mitochondrial functions together with Nrf1 Next, we aimed to identify transcription factors that cooperate with LSD1 in the control of OXPHOS gene expression. HOMER motif searches [25] revealed that promoter occupancy of LSD1 significantly correlates with the presence of binding sites for the transcription factor Nrf1 ( Fig. 3a ). To investigate whether LSD1 and Nrf1 are present in the same protein complex, differentiated 3T3-L1(LSD1) and 3T3-L1(Ctrl) adipocytes were subjected to sucrose gradient centrifugation. Western blot analysis showed that Nrf1 co-fractionates with LSD1 in both 3T3-L1(LSD1) and 3T3-L1(Ctrl) cells ( Fig. 3b ). In addition, co-immunoprecipitation with anti-LSD1 antibody confirmed the interaction between LSD1 and Nrf1 in 3T3-L1(LSD1) adipocytes ( Fig. 3c ). Furthermore, we identified the Nrf1 gene among the prominent direct LSD1 targets ( Supplementary Fig. 6a,b ). Accordingly, qRT–PCR and western blot analyses verified that elevated LSD1 levels resulted in increased Nrf1 transcript and protein levels ( Fig. 3d and Supplementary Fig. 6c,d ). 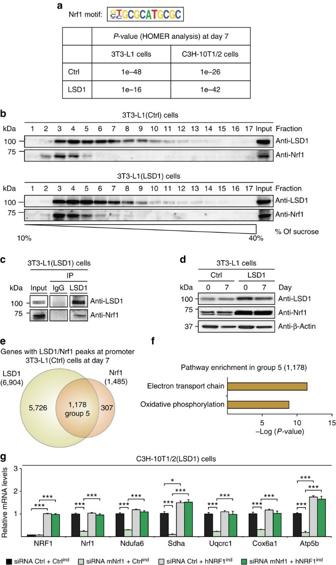Figure 3: LSD1 controls OXPHOS through Nrf1. (a) HOMER motif analysis of LSD1 ChIP-seq data unravel Nrf1 binding sites among the top scoring motifs. (b) Cell lysates from 3T3-L1(Ctrl) and 3T3-L1(LSD1) differentiated adipocytes were subjected to sucrose gradient centrifugation. Aliquots of the gradient fractions and total cell lysate (Input) were subjected to immunoblot analysis for LSD1 and Nrf1. (c) Co-immunoprecipitation of LSD1 and Nrf1 in differentiated 3T3-L1(LSD1) cells. Western blots were probed with the indicated antibodies. (d) Western blot analysis of LSD1 and Nrf1 expression in 3T3-L1(Ctrl) and 3T3-L1(LSD1) cells at indicated days. β-Actin served as a loading control. (e) Venn diagram depicting the number of genes with LSD1 and Nrf1 peaks at the promoter in differentiated 3T3-L1(Ctrl) cells (day 7). (f) Enriched pathways obtained from GO term analyses for the indicated sets of genes. (g) Relative transcript levels of the indicated markers in differentiated C3H-10T1/2(LSD1) cells transfected with unrelated control siRNA (siRNA Ctrl) or siRNA directed against mouseNrf15′ untranslated region (siRNA mNrf1) and infected with inducible empty control vector (Ctrlind) or humanNRF1(hNRF1ind) lentivirus, treated with Doxycycline (Dox) at day 3 of differentiation. (b–d) and (g):n=9; s.d. represents+s.e.m. Experiment (g) was independently repeated at least three times in triplicate. Statistical analysis was performed using (a) HOMER analysis or (g) two-tailed Student’st-test. *P<0.05 and ***P<0.001. Figure 3: LSD1 controls OXPHOS through Nrf1. ( a ) HOMER motif analysis of LSD1 ChIP-seq data unravel Nrf1 binding sites among the top scoring motifs. ( b ) Cell lysates from 3T3-L1(Ctrl) and 3T3-L1(LSD1) differentiated adipocytes were subjected to sucrose gradient centrifugation. Aliquots of the gradient fractions and total cell lysate (Input) were subjected to immunoblot analysis for LSD1 and Nrf1. ( c ) Co-immunoprecipitation of LSD1 and Nrf1 in differentiated 3T3-L1(LSD1) cells. Western blots were probed with the indicated antibodies. ( d ) Western blot analysis of LSD1 and Nrf1 expression in 3T3-L1(Ctrl) and 3T3-L1(LSD1) cells at indicated days. β-Actin served as a loading control. ( e ) Venn diagram depicting the number of genes with LSD1 and Nrf1 peaks at the promoter in differentiated 3T3-L1(Ctrl) cells (day 7). ( f ) Enriched pathways obtained from GO term analyses for the indicated sets of genes. ( g ) Relative transcript levels of the indicated markers in differentiated C3H-10T1/2(LSD1) cells transfected with unrelated control siRNA (siRNA Ctrl) or siRNA directed against mouse Nrf1 5′ untranslated region (siRNA mNrf1) and infected with inducible empty control vector (Ctrl ind ) or human NRF1 (hNRF1 ind ) lentivirus, treated with Doxycycline (Dox) at day 3 of differentiation. ( b – d ) and ( g ): n =9; s.d. represents+s.e.m. Experiment ( g ) was independently repeated at least three times in triplicate. Statistical analysis was performed using ( a ) HOMER analysis or ( g ) two-tailed Student’s t -test. * P <0.05 and *** P <0.001. Full size image To investigate the coordinated action of LSD1 and Nrf1 in OXPHOS gene regulation, we performed ChIP-seq analysis and established the genome-wide binding pattern of Nrf1 in 3T3-L1 cells. At day 7 of differentiation, 1,629 Nrf1 peaks were observed with 91% located at the promoter of 1,485 genes ( Fig. 3e and Supplementary Fig. 6e ). We found that the majority of Nrf1 target genes (1,178 out of 1,485, 79%) were also bound by LSD1 (group 5, Fig. 3e ). Pathway analysis for these genes revealed ‘electron transport chain’ and ‘OXPHOS’ among the top scoring pathways ( Fig. 3f ) as exemplified in Supplementary Fig. 6f . To further characterize the impact of the interaction between LSD1 and Nrf1 on oxidative capacities of adipocytes, we first transfected 3T3-L1(LSD1) or C3H-10T1/2(LSD1) cells with siRNA directed against Nrf1. siRNA-mediated knockdown of Nrf1 in LSD1-overexpressing cells significantly decreased expression of representative genes of the mitochondrial electron transport chain ( Supplementary Fig. 6g,h ). This effect could be rescued by lentivirus-mediated expression of RNA interference-resistant human NRF1 ( Fig. 3g ). Together, these data show that LSD1 promotes mitochondrial respiratory properties of fat cells, not only by inducing expression of but also in cooperation with Nrf1. LSD1 is essential for initiation of adipogenesis Pathway analyses unravelled a significant enrichment of ‘adipogenesis’ genes in both control and LSD1-overexpressing adipocytes ( Fig. 2c,d ). In line with this observation, it was previously reported that knockdown of LSD1 blocks differentiation of 3T3-L1 and C3H-10T1/2 cells [9] . We wondered whether LSD1, although required at early stages of adipogenesis, might be dispensable for terminal differentiation.To address this question, we engineered a conditional LSD1 allele by flanking exon 1 with loxP sites and deleted LSD1 by crossing mice harbouring the conditional allele to Rosa26-CreER T2 inducible deleter strain ( LSD1 Rosa26-CreERT2 ). Adipocyte precursors of the stromal-vascular fraction (SVF) from LSD1 Rosa26-CreERT2 mice were fluorescence-activated cell (FACS) sorted and treated with tamoxifen (Tam) or vehicle before or after induction of adipogenesis ( Supplementary Fig. 7a,b ). Loss of LSD1 by treatment with Tam 5 days before differentiation precluded expression of markers of mature adipocytes as well as accumulation of lipid droplets ( Fig. 4 ). On the opposite, treatment with Tam after day 3 of differentiation did not affect terminal adipogenesis ( Fig. 4 ), demonstrating that LSD1 is dispensable for induction of late adipogenic markers and lipid droplet accumulation. 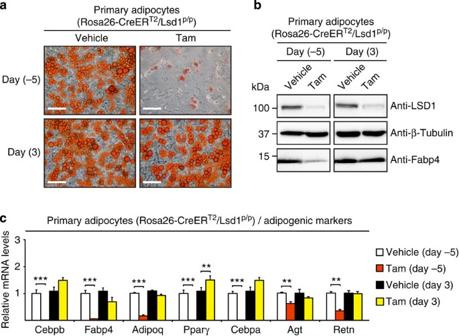Figure 4: LSD1 is essential for early adipogenesis, but dispensable at later stages of differentiation. (a) Oil red O staining (magnification: × 200; scale bar, 100 μm). (b) Western blot analysis of LSD1 and Fabp4, and (c) relative transcript levels of adipogenic markers in differentiated primary adipocytes from Rosa26-CreERT2/Lsd1p/pmice treated with Tamoxifen (Tam) or vehicle at the indicated time points of differentiation. β-Tubulin served as a loading control. (a–c):n=9; s.d. represents+s.e.m. Experiments (a,c) were independently repeated at least three times in triplicate. Statistical analysis was performed using two-tailed Student’st-test. **P<0.01 and ***P<0.001. Figure 4: LSD1 is essential for early adipogenesis, but dispensable at later stages of differentiation. ( a ) Oil red O staining (magnification: × 200; scale bar, 100 μm). ( b ) Western blot analysis of LSD1 and Fabp4, and ( c ) relative transcript levels of adipogenic markers in differentiated primary adipocytes from Rosa26-CreER T2 /Lsd1 p/p mice treated with Tamoxifen (Tam) or vehicle at the indicated time points of differentiation. β-Tubulin served as a loading control. ( a – c ): n =9; s.d. represents+s.e.m. Experiments ( a , c ) were independently repeated at least three times in triplicate. Statistical analysis was performed using two-tailed Student’s t -test. ** P <0.01 and *** P <0.001. Full size image To determine whether the impact of LSD1 on adipogenesis is dependent on its demethylase activity, primary adipocytes, 3T3-L1 and C3H-10T1/2 cells were treated with the LSD1-specific inhibitor GSK690 or vehicle ( Fig. 5a ). Similar to what we observed on knockout of LSD1 , treatment with LSD1 inhibitor before differentiation abolished adipogenesis, whereas treatment 3 days after induction of differentiation had no detectable effect ( Fig. 5b–f ). Together, these data show that catalytically active LSD1 is essential for early but not late adipogenesis. 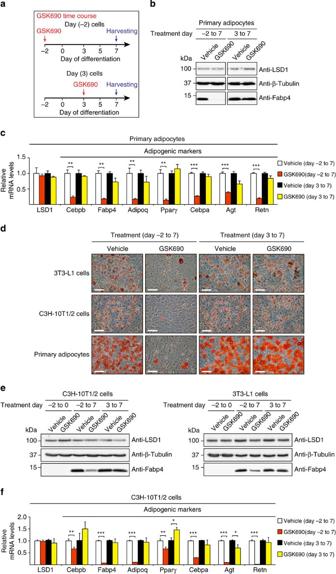Figure 5: LSD1 demethylase activity is essential for early adipogenesis but dispensable at later stages of differentiation. (a) Time scale of treatment of primary adipocytes, C3H-10T1/2, or 3T3-L1 cells with LSD1-specific inhibiter GSK690. (b) Western blot analysis of LSD1 and Fabp4 of differentiated primary adipocytes treated with LSD1-specific inhibiter GSK690 or vehicle at the indicated time points of differentiation. β-Tubulin served as a loading control. (c) Relative transcript levels of indicated markers in differentiated primary adipocytes treated with LSD1-specific inhibiter GSK690 or vehicle at the indicated time points of differentiation. (d) Oil red O staining of 3T3-L1, C3H-10T1/2, or differentiated primary adipocytes treated with LSD1-specific inhibiter GSK690 or vehicle at the indicated time points of differentiation. Magnification: × 200; scale bar, 100 μm. (e) Western blot analysis of LSD1 and Fabp4 of (left panel) C3H-10T1/2 or (right panel) 3T3-L1 cells treated with LSD1-specific inhibiter GSK690 or vehicle at the indicated time points of differentiation. β-Tubulin served as a loading control. (f) Relative transcript levels of the indicated markers in C3H-10T1/2 treated with LSD1-specific inhibiter GSK690 or vehicle at the indicated time points of differentiation. (b–f):n=9; s.d. represents+s.e.m. Experiments (c,f) were independently repeated at least three times in triplicate. Statistical analysis was performed using two-tailed Student’st-test. *P<0.05, **P<0.01 and ***P<0.001. Figure 5: LSD1 demethylase activity is essential for early adipogenesis but dispensable at later stages of differentiation. ( a ) Time scale of treatment of primary adipocytes, C3H-10T1/2, or 3T3-L1 cells with LSD1-specific inhibiter GSK690. ( b ) Western blot analysis of LSD1 and Fabp4 of differentiated primary adipocytes treated with LSD1-specific inhibiter GSK690 or vehicle at the indicated time points of differentiation. β-Tubulin served as a loading control. ( c ) Relative transcript levels of indicated markers in differentiated primary adipocytes treated with LSD1-specific inhibiter GSK690 or vehicle at the indicated time points of differentiation. ( d ) Oil red O staining of 3T3-L1, C3H-10T1/2, or differentiated primary adipocytes treated with LSD1-specific inhibiter GSK690 or vehicle at the indicated time points of differentiation. Magnification: × 200; scale bar, 100 μm. ( e ) Western blot analysis of LSD1 and Fabp4 of (left panel) C3H-10T1/2 or (right panel) 3T3-L1 cells treated with LSD1-specific inhibiter GSK690 or vehicle at the indicated time points of differentiation. β-Tubulin served as a loading control. ( f ) Relative transcript levels of the indicated markers in C3H-10T1/2 treated with LSD1-specific inhibiter GSK690 or vehicle at the indicated time points of differentiation. ( b – f ): n =9; s.d. represents+s.e.m. Experiments ( c , f ) were independently repeated at least three times in triplicate. Statistical analysis was performed using two-tailed Student’s t -test. * P <0.05, ** P <0.01 and *** P <0.001. Full size image To validate these observations in vivo , we crossed mice harbouring the conditional LSD1 allele to the well-established aP2-Cre deleter strain, which was initially described to mediate Cre recombination specifically in WAT and BAT [26] ( LSD1 aP2-Cre , Supplementary Fig. 8a,b ). Of importance for this study, Cre activity was recently reported to be not restricted to mature adipocytes, but was also observed in white and brown adipocyte precursors [27] . LSD1 aP2-Cre mice showed a complete absence of white fat pads ( Supplementary Fig. 8a ). These data confirm that in vivo LSD1 is essential for the development of WAT. Recently, Hino et al . [10] reported that knockdown of LSD1 increased OXPHOS in 3T3-L1 or C3H-10T1/2 cells. This observation appears to contradict our data showing an increase in OXPHOS on increased LSD1 expression. Of note, Hino et al . [10] investigated changes in OXPHOS on LSD1 depletion before induction of adipogenesis. Given the essential role of LSD1 during early adipogenesis observed by Musri et al . [9] in vitro and in this study, we hypothesized that the effects observed by Hino et al . [10] might be caused by the influence of LSD1 on adipocyte differentiation. To clarify this point, we performed a time-course experiment examining expression levels of differentiation markers and of mitochondrial activity in C3H-10T1/2 and 3T3-L1 cells treated with the LSD1-specific inhibitor GSK690 or vehicle. At day 0, we did not observe differences in mitochondrial activity (FL-2/FL-1 ratio) between cells treated with GSK690 or vehicle, showing that LSD1 inhibition does not alter OXPHOS in preadipocytes ( Supplementary Fig. 9a ). At days 1 and 7 of differentiation, we observed in vehicle-treated cells a gradual decrease in mitochondrial activity associated with the shift from energy consumption towards energy storage in differentiating C3H-10T1/2 and 3T3-L1 adipocytes ( Supplementary Fig. 9a ). Furthermore, differentiation was impaired in C3H-10T1/2 and 3T3-L1 cells treated with GSK690 as evidenced by decreased expression of adipogenic and white fat-specific markers such as Fabp4, Adipoq, Pparγ, Cebpa, Retn and Agt ( Supplementary Fig. 9b,c ). Importantly, owing to impaired differentiation, the decrease in mitochondrial activity was less pronounced in GSK690-treated C3H-10T1/2 and 3T3-L1 cells, and might be regarded as an increase relative to vehicle-treated cells ( Supplementary Fig. 9a ). Together, these observations suggest that impaired adipocyte differentiation hampers the analysis of a potential influence of LSD1 knockdown or inhibition on cellular metabolism at early time point of adipogenesis. Next, we asked whether LSD1 overexpression affects adipogenesis and thereby cellular metabolic activity. To address this point, we infected C3H-10T1/2 and 3T3-L1 cells with control (Ctrl) virus or lentivirus driving doxycycline-inducible expression of Flag-tagged LSD1 (LSD1 ind ) ( Supplementary Fig. 10a,b ). Induction of LSD1 2 days (day −2) before initiation of adipogenesis did not alter expression levels of adipogenic markers and lipid droplet accumulation compared with control cells ( Supplementary Figs 10c,d and 11a,b ). Importantly, induction of LSD1 3 days after initiation of differentiation was sufficient to induce oxidative metabolism ( Fig. 6a ) without affecting terminal differentiation ( Fig. 6b and Supplementary Fig. 11b ). Similarly, adipogenesis was not altered in 3T3-L1(LSD1) compared with 3T3-L1(Ctrl) cells ( Supplementary Fig. 11c,d ). Together, these data show that LSD1 overexpression does not affect adipogenesis and that an increase in LSD1 levels at later stages of adipocyte differentiation is sufficient to promote oxidative capacities. 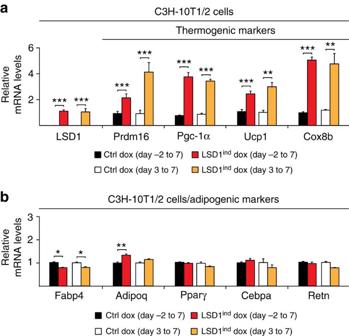Figure 6: LSD1 overexpression induces oxidative metabolism in adipocytes. (a,b) Relative transcript levels of the indicated markers in C3H-10T1/2 cells infected with control virus (Ctrl) or inducible LSD1 (LSD1ind) lentivirus, treated with Doxycycline (Dox) or vehicle at the indicated time points of differentiation. (a,b):n=9; s.d. represents+s.e.m. Experiments (a,b) were independently repeated at least three times in triplicate. Statistical analysis was performed using two-tailed Student’st-test. *P<0.05, **P<0.01 and ***P<0.001. Figure 6: LSD1 overexpression induces oxidative metabolism in adipocytes. ( a , b ) Relative transcript levels of the indicated markers in C3H-10T1/2 cells infected with control virus (Ctrl) or inducible LSD1 (LSD1 ind ) lentivirus, treated with Doxycycline (Dox) or vehicle at the indicated time points of differentiation. ( a , b ): n =9; s.d. represents+s.e.m. Experiments ( a , b ) were independently repeated at least three times in triplicate. Statistical analysis was performed using two-tailed Student’s t -test. * P <0.05, ** P <0.01 and *** P <0.001. Full size image LSD1 promotes oxidative capacities in WAT To investigate whether in vivo elevated levels of LSD1 have physiological functions comparable to those observed in tissue culture, we generated Tg mice expressing human LSD1 under the control of the Rosa26 promoter ( Supplementary Fig. 12a ). Western blotting, qRT–PCR and immunofluorescence analyses confirmed elevated LSD1 levels in WAT of Tg compared with control mice ( Supplementary Fig. 12b–d ). Histological analyses of WAT of Tg mice revealed the presence of islets of multilocular brown fat-like cells in epWAT and ingWAT ( Fig. 7a ). Ultrastructure analyses showed an increased number of hypotrophic lipid droplets, as well as dramatically elevated mitochondria size and number in Tg mice ( Fig. 7b,c and Supplementary Fig. 12e ). These findings were corroborated by an increased ratio between mitochondrial cytochrome C oxidase 2 ( Cox2 ) and nuclear fatty acid synthase ( Fasn ) DNA ( Supplementary Fig. 12f ). In addition, the activities of succinate dehydrogenase (Sdh, mitochondrial complex II) and Cox (mitochondrial complex IV) were significantly increased in WAT of Tg mice ( Fig. 7d ). Together, our observations demonstrate that elevated expression of LSD1 results in increased number and activity of mitochondria in WAT in vivo . In accordance with the data obtained in WAT, we observed decreased lipid droplet accumulation in BAT of Tg mice ( Fig. 7a ) together with increased expression levels of markers of oxidative metabolism and elevated activity of Sdh and Cox mitochondrial enzymes ( Supplementary Fig. 12g,h ). 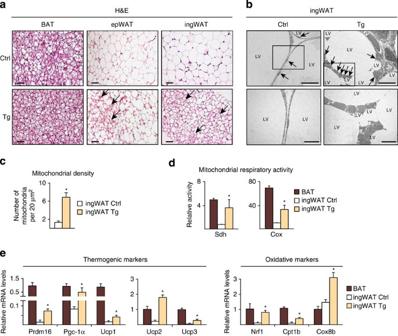Figure 7: Expression of LSD1 in transgenic mice induces oxidative capacities in WAT. (a) Haematoxylin and eosin staining (H&E) of interscapular BAT, epididymal (epWAT) and inguinal (ingWAT) WAT of control (Ctrl) and LSD1 transgenic (Tg) mice. Black arrows indicate beige fat islets. Scale bar, 100 μm. (b) Ultrastructure analysis of ingWAT of Ctrl and Tg mice. Black arrows indicate mitochondria. LV, lipid vesicle. Magnified regions are delimited by squares. Scale bars, 5 μm (upper panels) or 2 μm (lower panels). (c) Mitochondrial density determined from ultrastructure analysis of ingWAT of Ctrl and Tg mice. (d) Determination of Sdh (mitochondrial respiratory chain complex II) and Cox (mitochondrial respiratory chain complex IV) activities in ingWAT of Ctrl and Tg mice. BAT of Ctrl mice was used as a positive control. (e) Relative transcript levels of the indicated markers in ingWAT of Ctrl and Tg mice. (a,d,e):n=10, (b,c):n=5; s.d. represents+s.e.m. Experiments (d,e) were independently repeated at least three times in triplicate. Statistical analysis was performed using two-tailed Student’st-test. *P<0.05. Figure 7: Expression of LSD1 in transgenic mice induces oxidative capacities in WAT. ( a ) Haematoxylin and eosin staining (H&E) of interscapular BAT, epididymal (epWAT) and inguinal (ingWAT) WAT of control (Ctrl) and LSD1 transgenic (Tg) mice. Black arrows indicate beige fat islets. Scale bar, 100 μm. ( b ) Ultrastructure analysis of ingWAT of Ctrl and Tg mice. Black arrows indicate mitochondria. LV, lipid vesicle. Magnified regions are delimited by squares. Scale bars, 5 μm (upper panels) or 2 μm (lower panels). ( c ) Mitochondrial density determined from ultrastructure analysis of ingWAT of Ctrl and Tg mice. ( d ) Determination of Sdh (mitochondrial respiratory chain complex II) and Cox (mitochondrial respiratory chain complex IV) activities in ingWAT of Ctrl and Tg mice. BAT of Ctrl mice was used as a positive control. ( e ) Relative transcript levels of the indicated markers in ingWAT of Ctrl and Tg mice. ( a , d , e ): n =10, ( b , c ): n =5; s.d. represents+s.e.m. Experiments ( d , e ) were independently repeated at least three times in triplicate. Statistical analysis was performed using two-tailed Student’s t -test. * P <0.05. Full size image Consistent with the appearance of brown fat-like adipocytes in WAT of Tg mice, analyses of transcript and protein levels revealed significantly increased expression of thermogenic ( Prdm16 , Pgc-1α , Ucp1 , Ucp2 and Ucp3 ) and oxidative markers ( Nrf1 , Cpt1β and Cox8b ) ( Fig. 7e and Supplementary Fig. 13a,b ), whereas transcript and protein levels of adipogenic markers ( Fabp4 and Adipoq ) were not altered ( Supplementary Fig. 13b,c ). To investigate cell autonomy of LSD1 in Tg mice, adipocyte precursors from the SVF of Tg and control mice were isolated, FACS sorted and induced to undergo adipogenesis. Tg and control primary adipocyte cultures expressed equivalent levels of adipogenic markers during the path of differentiation ( Fig. 8a and Supplementary Fig. 14 ). In contrast, elevated levels of LSD1 in primary Tg adipocytes resulted in increased expression of thermogenic and oxidative markers ( Fig. 8a and Supplementary Fig. 14 ). Furthermore, adipocyte precursors from wild-type mice were isolated, FACS sorted and infected with control (Ctrl) or lentivirus driving doxycycline-inducible expression of Flag-tagged LSD1 ( Fig. 8b ). In full agreement with results obtained in C3H-10T1/2 and 3T3-L1 cells, we observed that also in primary adipocytes elevated LSD1 levels promoted the expression of oxidative markers without affecting adipogenesis ( Fig. 8b ). Taken together, these data demonstrate that in mice, LSD1 regulates oxidative capacities of adipocytes in a cell-autonomous manner. 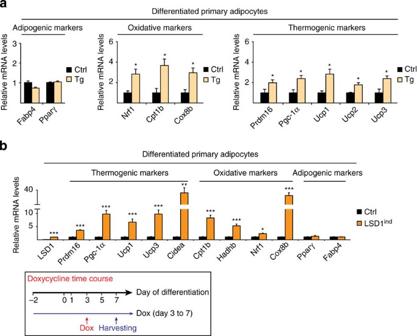Figure 8: LSD1 induces oxidative capacities in WAT in a cell-autonomous manner. (a) Relative transcript levels of the indicated markers in differentiated primary adipocytes from Ctrl and Tg mice. (b) Relative transcript levels of indicated genes in primary adipocytes infected with control virus (Ctrl) or inducible LSD1 (LSD1ind) lentivirus, treated with Dox or vehicle 3 days after the onset of differentiation. (a,b):n=9; s.d. represents+s.e.m. Experiments (a,b) were independently repeated at least three times in triplicate. Statistical analysis was performed using two-tailed Student’st-test. *P<0.05, **P<0.01 and ***P<0.001. Figure 8: LSD1 induces oxidative capacities in WAT in a cell-autonomous manner. ( a ) Relative transcript levels of the indicated markers in differentiated primary adipocytes from Ctrl and Tg mice. ( b ) Relative transcript levels of indicated genes in primary adipocytes infected with control virus (Ctrl) or inducible LSD1 (LSD1 ind ) lentivirus, treated with Dox or vehicle 3 days after the onset of differentiation. ( a , b ): n =9; s.d. represents+s.e.m. Experiments ( a , b ) were independently repeated at least three times in triplicate. Statistical analysis was performed using two-tailed Student’s t -test. * P <0.05, ** P <0.01 and *** P <0.001. Full size image LSD1 Tg mice are resistant to obesity and type-2 diabetes To investigate whether the presence of brown fat-like cells has physiological consequences, we subjected Tg mice on a high-fat diet (HFD) to metabolic analyses. During HFD feeding, Tg mice gained significantly less weight (~20%) than their control littermates ( Fig. 9a ). Body composition analyses assessed by quantitative nuclear magnetic resonance spectroscopy (qNMR) after 15 weeks of HFD showed that Tg animals had accumulated less fat, resulting in a higher lean/fat mass ratio compared with control mice ( Fig. 9b ). These data were corroborated by a decreased epWAT mass ( Supplementary Fig. 15a ). In accordance, histological analyses revealed adipocyte hypotrophy, as well as the presence of brown fat-like fat cells and increased Ucp1 levels in Tg mice ( Fig. 9c and Supplementary Fig. 15b ). The limited weight gain of Tg mice was not associated with decreased food intake ( Supplementary Fig. 15c ) or altered physical activity ( Supplementary Fig. 15d ). However, we observed higher energy expenditure as determined by oxygen consumption (VO 2 ) in Tg mice ( Fig. 9d ). CO 2 production (VCO 2 ) was not altered, resulting in a decreased respiratory quotient (RQ, VCO 2 /VO 2 ratio), showing a shift in fuel consumption from carbohydrate to fatty acid usage ( Fig. 9d ). Calorimetric parameters deduced from these analyses indicated that heat production was increased in Tg mice fed a HFD ( Supplementary Fig. 15e ). Taken together, these data show that Tg mice are less susceptible to obesity on a HFD due to increased energy expenditure. 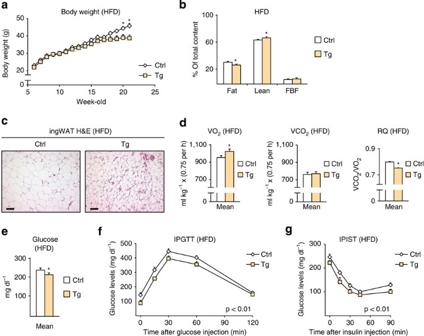Figure 9: Elevated LSD1 levels protect mice from HFD-induced obesity and type-2 diabetes. (a) Body weight of Ctrl and Tg mice fed a high-fat diet (HFD). (b) Fat, lean and free body fluid (FBF) content of Ctrl and Tg mice fed a HFD. (c) H&E staining of ingWAT of Ctrl and Tg mice fed a HFD. Scale bar, 200 μm. (d) VO2, VCO2and respiratory quotient (RQ) of Ctrl and Tg mice fed a HFD. (e) Serum glucose levels, (f) intraperitoneal glucose tolerance test (IPGTT) and (g) intraperitoneal insulin sensitive test (IPIST) of Ctrl and Tg mice fed a HFD. (a–g):n=10; s.d. represents+s.e.m. Statistical analysis was performed using two-tailed Student’st-test. *P<0.05. Figure 9: Elevated LSD1 levels protect mice from HFD-induced obesity and type-2 diabetes. ( a ) Body weight of Ctrl and Tg mice fed a high-fat diet (HFD). ( b ) Fat, lean and free body fluid (FBF) content of Ctrl and Tg mice fed a HFD. ( c ) H&E staining of ingWAT of Ctrl and Tg mice fed a HFD. Scale bar, 200 μm. ( d ) VO 2 , VCO 2 and respiratory quotient (RQ) of Ctrl and Tg mice fed a HFD. ( e ) Serum glucose levels, ( f ) intraperitoneal glucose tolerance test (IPGTT) and ( g ) intraperitoneal insulin sensitive test (IPIST) of Ctrl and Tg mice fed a HFD. ( a – g ): n =10; s.d. represents+s.e.m. Statistical analysis was performed using two-tailed Student’s t -test. * P <0.05. Full size image Diet-induced obesity is frequently associated with glucose intolerance and progressive metabolic dysfunction [28] . Notably, Tg mice on a HFD displayed decreased blood glucose levels ( Fig. 9e ), associated with improved glucose tolerance relative to control mice ( Fig. 9f ). Tg mice were also more insulin sensitive, as determined by insulin-sensitive test ( Fig. 9g ), showing that Tg mice are more resistant to HFD-induced type-2 diabetes. These observations show that increased LSD1 levels result in raised energy expenditure, which limits HFD-induced obesity and type-2 diabetes. LSD1 Tg mice are more reactive to β3-adrenergic signalling LSD1 levels are increased in mice on cold exposure or treatment with the β3-selective adrenergic agonist CL316,243 ( Fig. 1a,b ), and increased LSD1 levels suffice to promote thermogenesis and mitochondrial activity in WAT ( Fig. 7e ). Thus, we hypothesized that Tg mice with elevated LSD1 levels might be more reactive to cold exposure or treatment with β3-adrenergic agonist. As shown in Fig. 10a,b , the amount of brown-like fat cells and Ucp1 expression levels in WAT increased faster in Tg than in control mice during cold exposure. Moreover, treatment with CL316,243 resulted in more clusters of beige fat cells and Ucp1 protein expression in WAT of Tg compared with control mice ( Fig. 10c,d ). Accordingly, qRT–PCR analyses showed significantly increased expression of Prdm16 , Pgc-1α , Ucp1 , Cidea and Cpt1b in WAT of Tg mice on stimulation with the β3-adrenergic agonist due to their increased susceptibility for browning ( Fig. 10e ). 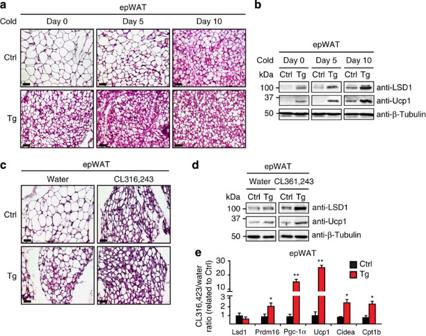Figure 10: LSD1 Tg mice are more sensitive to cold exposure. (a) Haematoxylin and eosin (H&E) staining, (b) western blot analysis of LSD1 and Ucp1 expression in mice exposed to cold for 0, 5, or 10 days. β-Tubulin was used as a loading control. (c) H&E staining, (d) western blot analysis of LSD1 and Ucp1, and (e) relative transcript levels of indicated genes of epWAT of Ctrl and Tg mice treated with vehicle or CL316,243. β-Tubulin was used as a loading control. Scale bars, 100 μm. (a–e):n=10; s.d.represents+s.e.m. Experiment (e) was independently repeated at least three times in triplicate. Statistical analysis was performed using two-tailed Student’st-test. *P<0.05 and **P<0.01. Figure 10: LSD1 Tg mice are more sensitive to cold exposure. ( a ) Haematoxylin and eosin (H&E) staining, ( b ) western blot analysis of LSD1 and Ucp1 expression in mice exposed to cold for 0, 5, or 10 days. β-Tubulin was used as a loading control. ( c ) H&E staining, ( d ) western blot analysis of LSD1 and Ucp1, and ( e ) relative transcript levels of indicated genes of epWAT of Ctrl and Tg mice treated with vehicle or CL316,243. β-Tubulin was used as a loading control. Scale bars, 100 μm. ( a – e ): n =10; s.d.represents+s.e.m. Experiment ( e ) was independently repeated at least three times in triplicate. Statistical analysis was performed using two-tailed Student’s t -test. * P <0.05 and ** P <0.01. Full size image In summary, our data demonstrate that LSD1 controls thermogenesis and oxidative metabolism of adipose tissue by increasing mitochondrial biogenesis and respiration via Nrf1, thus protecting mice against metabolic-related disorders. In this work we show that LSD1 expression is upregulated in WAT of mice on cold exposure or β3-adrenergic stimulation. Both stimuli are known to induce number and activity of mitochondria in WAT [18] , and several factors such as Prdm16 and Pgc-1α have been implicated in this metabolic adaptation [29] . Our results demonstrate that increased LSD1 expression is sufficient to enhance oxidative capacities of mature adipocytes. Thus, elevated LSD1 levels mimic the effects of cold exposure or β3-adrenergic treatment. LSD1-mediated metabolic adaptation is, to a large extent, due to promoting the expression of the vast majority of genes encoding subunits of the mitochondrial respiratory chain, and of Tfam, the major regulator of mitochondrial biogenesis [19] . Our genome-wide binding and transcriptome analyses demonstrate that LSD1 directly regulates these genes in cooperation with Nrf1. Nrf1 has been identified as a key factor controlling mitochondrial biogenesis and ATP production in several metabolic tissues, including WAT and skeletal muscle [22] , [30] . An interaction between LSD1 and Nrf1 was recently observed in MCF7 breast cancer cells [31] , but no physiological relevance of this interaction was reported. Altogether, these data suggest a more general mechanism by which LSD1 controls metabolic properties of cells in cooperation with Nrf1. In WAT of mice, transgenic expression of LSD1 induces the formation of functional islets of brown-like adipocytes. These islets express increased levels of uncoupling proteins, which uncouple O 2 consumption from ATP production to dissipate energy as heat. Accordingly, Tg mice exhibit higher body temperature than their control littermates, which limits their weight gain in response to a HFD. The reduced body weight of Tg mice leads to resistance to HFD-induced type-2 diabetes [28] , making LSD1 a potential target to treat obesity-related disorders. In previous reports, knockdown or inhibition of LSD1 has been reported to impair differentiation of 3T3-L1 preadipocytes [9] and to result in increased oxidative capacities [10] . Our data obtained in vitro and for LSD1 aP2-Cre mice confirm that LSD1 ablation during early stages of differentiation abolishes formation of mature adipocytes. In comparison, elevated LSD1 levels do not influence adipogenesis, but increase oxidative capacities of mature adipocytes. The seeming contradiction between increased oxidative capacities on LSD1 knockdown suggested by Hino et al . [10] and enhanced OXPHOS noticed on LSD1 overexpression can be explained by distinct effects of LSD1 knockdown or overexpression on adipocyte differentiation. On differentiation, we observe a reduction of mitochondrial activity in 3T3-L1 and C3H-10T1/2 cells, which is likely to reflect the shift of adipocyte metabolism from fuel consumption to energy storage. Thus, impaired differentiation of both cell lines due to inhibition of LSD1 partially prevents the decrease in mitochondria activity, which may be regarded as an increase when compared with differentiating control cells. Our observation that LSD1 protein levels increase in WAT of mice on cold exposure or β3-adrenergic stimulation suggests a regulatory mechanism that adapts LSD1 levels according to energy requirements imposed by the environment. Such a mechanism would help mice to survive cold season by mobilizing energy supplies and increasing adaptive thermogenesis. This hypothesis implies that in humans it may be possible to promote energy expenditure and treat obesity and metabolic syndrome by modulation of LSD1 expression or activity. Mouse studies All mice were housed in the pathogen-free barrier facility of the University Medical Center Freiburg in accordance with institutional guidelines and approved by the regional board. Mice were maintained in a temperature- and humidity-controlled animal facility with a 12-h light/dark cycle, free access to water and a standard rodent chow (Kliba, breeding, 3,807). The HFD study was carried out with a chow containing 4.056 kcal kg − 1 (fat: 1.600 kcal kg − 1 and sucrose: 1.600 kcal kg − 1 ; Research Diets). HFD was given to mice at 5 weeks of age. Male mice were analysed at 25 weeks of age. For cold exposure experiments, C57/Bl6N mice were maintained at 10 °C with a 12-h light/dark cycle, free access to water and a standard rodent chow. Animals were killed by cervical dislocation, tissues were immediately collected, weighted, frozen in liquid nitrogen or processed for further analyses. Nomenclature for dissected adipose depots was used according to Seale et al . [17] Epididymidal WAT (epWAT) is the prominent bilateral intra-abdominal visceral depots in male mice attached to the epididymis. Inguinal WAT (ingWAT) is the bilateral superficial inguinal depots between the skin and muscle fascia just anterior to the lower segment of the hind limbs. Interscapular BAT (BAT) is the most prominent depot of brown adipocytes in rodents, found between the scapulae. In vivo experiments including food consumption, serum analysis, glucose tolerance and insulin sensitivity tests (IPISTs), temperature measurements, body lean and fat contents, and energy expenditure were described [32] . CL316,243 (Sigma-Aldrich) was injected to C57/Bl6N mice intraperitoneally at 1 mg kg − 1 . Generation of Rosa26- LSD1 mutant transgenic mice To generate Tg mice, the complete human wild-type LSD1 complementary DNA was cloned 3′ to the Rosa26 promoter/enhancer ( Supplementary Fig. 12a ). Tg mice were generated by pronuclear injection into fertilized FVB oocytes. Mice were then backcrossed on a C57/Bl6N background. For analyses, wild-type littermates were used as controls. Mice were genotyped by PCR amplification of genomic DNA extracted from tail biopsies using the DirectPCR extraction kit (Viagen) with primers for detection of the transgene Rosa26- LSD1 ( Supplementary Table 1 ). Generation of conditional LSD1 knockout mice The targeting strategy for the conditional deletion of the first exon of LSD1 ( LSD1 tm1Schüle ) [33] is available on request. Briefly, a targeting vector was generated from genomic DNA. The pGK-Neo cassette was cloned between two FRT sites, and LoxP sites flanking exon 1 and pGK-Neo cassette were introduced by PCR-based site-directed mutagenesis. The resulting 10.5-kb fragment was electroporated into embryonic stem (ES) cells and G418 neomycin-resistant clones were expanded. Selected ES cells were injected into C57BL/6 blastocysts. Resulting mice were bred to Rosa26-Flp mice to delete the pGK-Neo fragment and obtain conditional LSD1 mice. To delete LSD1 , conditional LSD1 mice were crossed to aP2 -Cre mice [26] to selectively ablate LSD1 in adipose tissue. Mice were then backcrossed on a C57/Bl6N background. Homozygous conditional mice were used as controls. Mice were genotyped with primers for detection of the conditional LSD1 and the deleted alleles ( Supplementary Table 1 ). Analysis of mitochondrial activity Tissues obtained from mice were immediately frozen in liquid nitrogen. The activities of the respiratory chain enzyme complex II (Sdh) and complex IV (Cox) were determined as described [34] . Briefly, mitochondria were isolated in extraction medium (20 mM Tris, pH 7.2, 250 mM saccharose, 2 mM EGTA, 40 mM KCl and 1 mg.ml − 1 BSA). For Sdh activity measurements, samples were mixed with S medium (10 mM KH 2 PO 4 , 2 mM EDTA and 1 mg ml − 1 BSA, pH7.8), 8 μM rotenone, 40 μM dichlorophenolindophenol , 200 μM ATP, 320 μM KCN, 5 mM succinate and 16.5 μg ml − 1 decyl-ubiquinone. Decrease of absorbance is observed at 412 nm. For Cox activity measurements, samples were mixed with C+ medium (10 mM KH 2 PO 4 , 300 mM succrose and 1 mg ml − 1 BSA, pH6.5), 3.75 mM Lauryl maltoside and 14 μM cytochrome c reduced with dithionite crystals. Decrease of absorbance is observed at 550 nm. Food consumption Mice were individually housed. Food pellets (150 g) were delivered and weighed after 1 week. Weekly food consumption was calculated by subtracting the final from the initial pellet weight. Serum analysis Blood was collected from retro orbital sinus after a 6-h fast that started at the beginning of the light cycle. Glucose levels were determined on a drop of blood collected from the tail vein from mice after 6 h of fasting with an Accu-Chek Active blood glucometer (Roche, France) [35] . Glucose tolerance and IPISTs Intraperitoneal glucose tolerance test and IPIST were performed with mice fed a HFD after 16 or 6 h of fasting, respectively. For intraperitoneal glucose tolerance test, following measurement of the basal glucose level (time 0), mice were intraperitoneally injected with 20% glucose in sterile saline solution (0.9% NaCl) at a dose of 2 g glucose Per kg body weight. Blood was collected from the tail vein after 15, 30, 45, 60, 90 and 120 min for glucose determination. For IPIST, mice were intraperitoneally injected with porcine insulin (0.5 U kg − 1 ; Sigma). Blood was collected at 15, 30, 60 and 90 min. Body lean and fat content Body lean and fat content were recorded in anaesthetized mice by qNMR (PIXIMUS, GE Medical Systems) according to the manufacturer’s instructions. The study was performed at the Mouse Clinical Institute (Illkirch, France). Energy expenditure Total activity, oxygen consumption (O 2 ) and carbon dioxide (CO 2 ) production were measured with a LabMaster (TSE systems) at 26 min intervals for 24 h. VO 2 and VCO 2 values were normalized to body mass. The RQ corresponds to VCO 2 /VO 2 . Heat (cal h − 1 ) was calculated using the formula: Heat (H)=(Caloric Value × VO 2 × 0.001)/body weight × 0.75 (Caloric Value=3.815+1.232 × RQ). Body temperature was measured with a rectal probe linked to a digital thermometer (Bioseb). Histological and immunofluorescence analysis Tissues were fixed in 10% buffered formalin and embedded in paraffin. For immunofluorescence analyses, 5 μm paraffin sections were deparaffinized, rehydrated, boiled in antigen unmasking solution (Vector Laboratories, H-3300) for 10 min, cooled to room temperature, washed three times with PBS, 0.1% Triton-X100 for 5 min, incubated for 1 h in 5% fetal bovine serum (FBS; Gibco, 10270-106) in PBS, 0.1% Triton-X100, followed by overnight incubation at 4 °C with anti-LSD1 (ref. 1 ) (1/1,000) antibody. Slides were then incubated with secondary antibody conjugated to Alexa546 (Invitrogen, 1/400) and mounted in aqueous medium (Fluoromount-G, SouthernBiotech, 0100-01) with DAPI (4',6-diamidino-2-phenylindole; Sigma, D-9542, 1/1,000). Between each step, sections were washed with PBS, 0.1% Triton-X100. For ultrastructural analyses, samples were fixed by immersion in 2.5% glutaraldehyde and 2.5% paraformaldehyde in cacodylate buffer (0.1 M, pH 7.4), washed in cacodylate buffer for 30 min and kept at 4 °C. Post-fixation was performed with 1% osmium tetraoxide in 0.1 M cacodylate buffer for 1 h at 4 °C and dehydration through graded alcohol (50, 70, 90 and 100%) and propylene oxide for 30 min each. Samples were embedded in Epon 812. Ultrathin sections were cut at 70 nm and contrasted with uranyl acetate and lead citrate and examined at 70 kV with a Morgagni 268D electron microscope. Images were captured digitally by a Mega View III camera (Soft Imaging System). Mitochondria number and cross-section areas were determined with the Image J software (NIH). RNA preparation and analysis RNA was isolated with TRIzol Reagent (Invitrogen). Two micrograms of RNA were converted to cDNA with SuperScript II reverse transcriptase (Invitrogen) and polyT oligonucleotides according to the supplier’s protocol. qRT–PCR was performed using the Abgene SYBR Green PCR kit (Invitrogen) according to the supplier’s protocol. Data were analysed using the standard curve method [36] . 36b4 , Hprt , or Tbp were used for normalization. Primer sequences are given in Supplementary Table 2 . RNA sequencing RNA samples were sequenced by the standard Illumina protocol to create raw sequence files (.fastq files). We aligned these reads to the mm10 build of the mouse genome using TopHat version 2 (ref. 37 ). The aligned reads were counted with the homer software (analyse RNA) and DEG’s were identified using EdgeR [38] and DESeq version 1.8.3 (ref. 39 ). Western blot analysis and co-immunoprecipitation assays Experiments were performed as described [1] . Fat tissues were grounded in RIPA buffer (50 mM Tris, pH 7.5, 1% NP40, 0.5% sodium deoxycholate, 0.1% SDS, 150 mM NaCl, 5 mM EDTA and protease inhibitor cocktail (45 μg ml −1 , Roche, 11 873 580 001)) at 4 °C. Homogenates were separated in 10% polyacrylamide gels and blotted to Hybond nitrocellulose membranes (GE Healthcare). Membranes were decorated using the following antibodies: anti-LSD1 (ref. 1 ) (1/1,000), anti-Prdm16 (Abcam, ab118573, 1/500), anti-Ucp1 (Abcam, ab10983, 1/1,000), Fabp4 (Santa-Cruz, sc-18661, ½,000), anti-Nrf1 (Abcam, ab55744, 1/1,000), anti-Flag (Sigma, F3165, 1/500), anti-β-Tubulin (Sigma, T6074, 1/10,000), or anti-β-Actin (Sigma, A1978, 1/10,000). Secondary antibodies conjugated to horseradish peroxidase (GE Healthcare) were detected using an enhanced chemiluminescence detection system (GE Healthcare). Protein levels were quantified using the Chemi Capt software (Peqlab). Uncropped scans are available in Supplementary Fig. 16 . Sucrose density centrifugation Sucrose was dissolved in 50 mM Tris, 100 mM NaCl and Complete Protease Inhibitor (EDTA-free, Roche). Whole-cell lysate was added to the 40–10% sucrose gradient and centrifuged at 185,000 g for 16 h. Seventeen fractions were collected and immunoblotted with the indicated antibodies. ChIP sequencing ChIP experiments were performed using anti-LSD1 (20,752, Schüle Laboratory) or anti-Nrf1 (Abcam, ab55744, lot GR 95770-1) antibodies, on protein A-Sepharose 4B (GE Healthcare) essentially as described [40] . Libraries were prepared from immunoprecipitated DNA according to standard methods. ChIP-seq libraries were sequenced using a HiSeq 2000 (Illumina) and mapped to the mm10 reference genome using bowtie 2 (ref. 41 ). Data were further analysed using the peak finding algorithm MACS 1.41 (ref. 42 ) using input as control. All peaks with false discovery rate>1% were excluded from further analysis. The uniquely mapped reads were used to generate the genome-wide intensity profiles, which were visualized using the IGV genome browser [43] . HOMER [25] was used to annotate peaks, to calculate overlaps between different peak files, and for motif searches. The genomic features (promoter, exon, intron, 3′ untranslated region and intergenic regions) were defined and calculated using Refseq and HOMER. Genes annotated by HOMER were further used for a pathway analysis [25] . Quantification of mitochondrial and nuclear DNA Fat pads were digested overnight with Proteinase K and DNA was extracted with phenol–chloroform. Mitochondrial and nuclear DNA was amplified by quantitative PCR using Cox2 and Fasn primers ( Supplementary Table 2 ), respectively. Plasmids The following plasmids were used: pLenti4_Flag_HA_Puro and pLenti4_Flag_HA_Puro_LSD1, pSlik-Neo, pSlik-Neo_Flag-HA_LSD1 and pSlik-Neo_Flag-HA_NRF1. Plasmids were obtained by Gateway LRII cloning in pLenti4 vector (Invitrogen) or in a puromycin-selectable and doxycycline-inducible pSlik-Neo plasmid. Cloning details can be obtained on request. Adipocyte precursor isolation and flow cytometry Epididymal and inguinal fat pads were cut in small pieces and incubated with 1 mg ml −1 collagenase I for 40 min [44] , [45] . The cell suspension was filtered through a 150-μm nylon mesh and the SVF was isolated by low-speed centrifugation. For FACS analysis, erythrocyte-free SVF cells were incubated with a mix of antibodies against different surface markers as described previously [46] (anti-Ter119 fluorescein isothiocyanate (FITC), eBioscience, 11–5921, 0.5 mg ml − 1 ; anti-Cd45, FITC, eBioscience, 11–0451, 0.5 mg ml − 1 ; anti-Cd31 FITC, eBioscience, 11–0311, 0.5 mg ml − 1 ; anti-Sca1 PE/Cy7, BioLegend/Biozol, 122514, 1/500; and anti-Cd34 PE, Abcam, ab23830, 1/250) and sorted using an Aria flow cytometer (BD Biosciences). Dead cells were removed using DAPI staining (1/10,000). Cells negative for Ter119, Cd45 and Cd31, and positive for both Sca1 and Cd34 were considered as adipocyte precursor cells. Primary adipocytes were cultured in DMEM/F12 containing 10% FBS. Cell culture Mouse 3T3-L1 (ATCC, CL-173) and C3H-10T1/2, Clone 8 (ATCC, CCL-226) preadipocytes were maintained in DMEM or Eagle’s minimal essential medium, respectively, supplemented with 10% FBS and glutamine. Differentiation of primary adipocytes, 3T3-L1, and C3H-10T1/2 cells was induced by treatment of confluent cells (designated day 0) with an adipogenic mixture consisting of 10 μg ml − 1 insulin (Gibco), 1 μM dexamethasone (Calbiochem), 10 μM rosiglitazone (Cayman) and 500 μM isobutylmethylxanthine (Serva) in the presence of 10% FBS. The differentiation medium was replaced 3 days later (day 3) with medium supplemented with 10% FBS and 10 μg ml − 1 insulin for 2 days. Subsequently, the cells were cultured in the same medium for 2 more days (day 7). For the determination of mitochondrial metabolism, cells were stained with fluorescent dye JC-1 (Invitrogen) followed by flow cytometric analysis. Following trypsin treatment, cells were exposed to 2 μM of JC-1 in culture medium for 30 min at 37 °C and suspended in PBS for FACS analysis. Green and red fluorescent signals corresponding to mitochondrial mass (FL-1) and mitochondrial membrane potential (FL-2), respectively, were detected using a FACS Canto cytometer (Becton Dickinson). 3T3-L1 and C3H-10T1/2 preadipocytes were infected with pLenti4_Flag_HA_Puro, pLenti4_Flag_HA_Puro_LSD1, pSlik-Neo, pSlik-Neo_LSD1, or pSlik-Neo_NRF1 virus, and subsequently selected in medium containing 1 μM puromycin (Sigma) or 500 μM geneticin (G-418, GibcoBRL). LSD1 inhibiter GSK690 was applied 2 days before differentiation. Differentiated 3T3-L1 or C3H-10T1/2 cells were treated with CL316,243 at 1 μM for 4 h. 3T3-L1 or C3H-10T1/2 cells were treated with BMP7 before differentiation at 50 nM for 48 h. 3T3-L1 cells or C3H-10T1/2 were transfected with 1 μM siRNA against LSD1, Nrf1 or unrelated control (Invitrogen) using DharmaFECT 1 or 2 (Thermo Scientific), respectively, according to the manufacturer’s instructions. siRNA oligonucleotide sequences were as follows: LSD1 siRNA: 5′-CCCAAAGAUCCAGCUGACGUUUGAA-3′; Control LSD1 siRNA: 5′-UUCUUAGCAAGACUGGUCUCUAGGG-3′; Nrf1 siRNA (5′ untranslated region): 5′-UCGAAUGGUAUGUGGUUCAUGUAGA-3′; Nrf1 siRNA (ORF): 5′-UAUGGUAGCCAUGUGUUCAGUUUGG-3′; Control siRNA: 5′-UAUUUGGAUGUACCUGUGGACUUGG-3′. Data analysis Data are represented as mean+s.e.m. Significance (except Fig. 3a ) was calculated by a two-tailed Student’s t -test. How to cite this article: Duteil, D. et al . LSD1 promotes oxidative metabolism of white adipose tissue. Nat. Commun. 5:4093 doi: 10.1038/ncomms5093 (2014). Accession codes: ChIP-Seq and RNA-seq data have been deposited in Gene Expression Omnibus under accession code GSE50934 .